Sphingosine-1-phosphate promotes expansion of cancer stem cells via S1PR3 by a ligand-independent Notch activation Many tumours originate from cancer stem cells (CSCs), which is a small population of cells that display stem cell properties. However, the molecular mechanisms that regulate CSC frequency remain poorly understood. Here, using microarray screening in aldehyde dehydrogenase (ALDH)-positive CSC model, we identify a fundamental role for a lipid mediator sphingosine-1-phosphate (S1P) in CSC expansion. Stimulation with S1P enhances ALDH-positive CSCs via S1P receptor 3 (S1PR3) and subsequent Notch activation. CSCs overexpressing sphingosine kinase 1 (SphK1), an S1P-producing enzyme, show increased ability to develop tumours in nude mice, compared with parent cells or CSCs. Tumorigenicity of CSCs overexpressing SphK1 is inhibited by S1PR3 knockdown or S1PR3 antagonist. Breast cancer patient-derived mammospheres contain SphK1 + /ALDH1 + cells or S1PR3 + /ALDH1 + cells. Our findings provide new insights into the lipid-mediated regulation of CSCs via Notch signalling, and rationale for targeting S1PR3 in cancer. Growing evidence suggests that many types of cancer, including breast, lung and prostate cancer, are initiated from a small population of cancer stem cells (CSCs; also called tumour-initiating cells) [1] , [2] , [3] , [4] , [5] , [6] , [7] , [8] . This minor population produces the bulk of cancers through continuous self-renewal and differentiation, which contributes to cancer heterogeneity. Therefore, it is essential to elucidate the signalling and regulatory mechanisms that are unique to CSCs, and to design novel therapeutic agents against CSCs. CSCs have been isolated from diverse tumours and established cell lines, using several methods encompassing cell surface markers, aldehyde dehydrogenase (ALDH) activity, side population (SP) and sphere-forming ability. ALDH assays rely on the fact that the level of ALDH, a detoxifying enzyme responsible for the oxidation of intracellular aldehydes, is higher in stem cells than in differentiated cells [4] . ALDH1 expression is correlated with poor clinical prognosis in various cancers, such as breast, lung and prostate cancer [4] , [5] , [6] . Because CSCs have been considered to have molecular similarities to embryonic and normal adult stem cells, the self-renewal behaviour of CSCs has been reported to be mediated by several signalling pathways, such as Notch, Hedgehog and Wnt [9] . However, the molecular mechanisms that regulate the frequency and maintenance of CSCs via self-renewal signals remain poorly understood. Autocrine and paracrine signalling plays a key role in maintaining the stem cell state and expansion of stem cells [10] . We therefore speculated that receptors for autocrine/paracrine factors might play a key role in CSC regulation. Using microarray screening in an ALDH-positive cell population of human breast cancer MCF-7 cells, we found that several receptors are upregulated. Among them, on the basis of pathophysiological properties, we focused on S1P receptor 3 (S1PR3), a receptor for a lipid mediator sphingosine-1-phospahate (S1P). S1P is known to exert multiple responses, such as proliferation, survival and cytoskeletal rearrangement, via its G protein-coupled receptor (GPCR) in many cell types [11] . S1P is synthesized from sphingosine by sphingosine kinase (SphK); two isoforms of mammalian SphK (sphingosine kinase 1 (SphK1) and SphK2) have been cloned and characterized [12] , [13] . In addition, the SphK1/S1P pathway has also been implicated in tumour progression [14] , [15] . S1P has also been shown to accumulate in the tumour microenvironment [16] . Although lipid mediators in cancer have been studied extensively, the role(s) of SphK1/S1P in CSCs remain unclear. We demonstrate here that S1P regulates expansion of CSCs in several types of cancer. Our findings suggest that Notch activation is essential for S1P-induced proliferation of CSCs via S1PR3. We show that SphK1 regulates the tumorigenicity of breast CSCs via S1PR3. Using clinical samples, we show that breast cancer patient-derived CSCs contain SphK1 + /ALDH1 + cells or S1PR3 + /ALDH1 + cells. Thus, these results implicate the S1P signalling pathway as therapeutic targets in CSCs. S1P is a regulator of CSC population via S1PR3 We used an ALDH assay system to study the signalling pathways that regulate the frequency and maintenance of CSCs. Many cancer cell lines, including oestrogen receptor-positive MCF-7 cells, are known to contain an ALDH-positive cell population [5] , [6] , [17] , [18] . Consistent with a previous report [4] , we confirmed that ALDH-positive cell population in MCF-7 cells possessed CSC-like properties, as assessed by expression of stem cell markers, drug resistance and tumorigenicity ( Supplementary Fig. 1 ). Through microarray analysis, we investigated a possible receptor that increases the proportion of the ALDH-positive cell population in MCF-7 cells as a CSC model. We found S1PR3 as a possible candidate in CSC regulation ( Supplementary Data 1 ). S1PR3 was highly expressed in the ALDH-positive cell population, a finding confirmed by quantitative polymerase chain reaction (qPCR) assays ( Fig. 1a ). S1PR2 expression was lower in the ALDH-positive cell population compared with MCF-7 cells, and other types of S1PR are yet to be detected in MCF-7 cells ( Supplementary Fig. 2 ) [19] , [20] . Stimulation with S1P increased the proportion of ALDH-positive cell population in a dose-dependent manner, with a maximal response observed at 100 nM ( Fig. 1b ). Similar to S1P, dihydro-S1P, another S1PR3 ligand, also increased the ALDH-positive cell population ( Supplementary Fig. 3 ). Moreover, stimulation with S1P increased the number of SP cells ( Fig. 1c ), mammosphere-forming efficiency ( Fig. 1d ), CD44 + /CD24 − population ( Fig. 1e ) and expression of stem cell markers ( Fig. 1f ). These data indicate that stimulation with S1P leads to an increase in breast CSCs. In contrast, lysophosphatidic acid (LPA), another well-studied lipid mediator, did not increase CSCs in MCF-7 cells. To confirm the involvement of S1PR3, we inhibited S1PR3 using pharmacological antagonists and RNA interference techniques. The effects of S1P were blocked by the S1PR3 antagonist TY52156 (ref. 21 ). Another antagonist CAY10444, which is structurally different from TY52156, also inhibited the S1P effect. In contrast, the S1PR2 antagonist JTE013 had little effect ( Fig. 1g ). Experiments using small interfering RNAs (siRNA) confirmed the effects of antagonists ( Fig. 1h ). In addition, short hairpin RNAs (shRNAs) against S1PR3 also inhibited the enhancement of mammosphere-forming ability by S1P ( Supplementary Fig.4 ). Similar results with ALDH assay were obtained in triple-negative MDA-MB-231 cells ( Supplementary Fig. 5a,b ), suggesting that S1P regulates both luminal and triple-negative type of breast CSCs. Furthermore, we examined CSCs from other tumour types to determine whether these effects of S1P are limited to breast cancer cell lines. Similar to MCF-7 cells, stimulation with S1P increased the ALDH-positive cell population in human lung cancer A549 cells, human prostate cancer LNCaP cells, human glioma U251MG cells and human ovarian cancer OVCAR-5 cells ( Supplementary Fig. 6a ). In addition, TY52156 inhibited the S1P effect in these cell lines. Taken together, these data demonstrate that S1P has an ability to increase the number of CSCs via S1PR3 in several types of cancer. 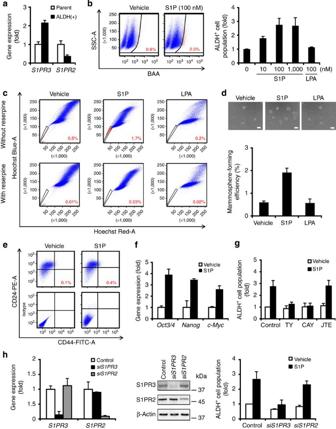Figure 1: Role of S1PR3 in the ALDH-positive cell population within the MCF-7 cell line. (a) Expression levels of S1PR (S1PR2andS1PR3) in parental or ALDH-positive MCF-7 cells by qPCR. Data represent mean±s.d. (n=3). (b) Representative flow data with ALDH substrate in the presence or absence of S1P (100 nM, 3 days) in MCF-7 cells. Dose-dependent effects of S1P in the proportion of ALDH-positive cell population. Data represent mean±s.d. (n=3). (c) Representative flow data of the SP assay with Hoechst 33342 dye alone or in the presence of reserpine (15 μg ml−1). (d) Effects of S1P (100 nM) on mammosphere-forming efficiency in MCF-7 cells. The number of mammospheres was microscopically counted and the percentage of mammosphere-forming cells was determined as mammosphere-forming efficiency (%). The scale bar, 100 μm. Data represent mean±s.d. (n=3). (e) Effects of S1P (100 nM) on CD44+/CD24−population in MCF-7 cells. (f) Effects of S1P (100 nM) on expression of stem cell markers by qPCR. Data represent mean±s.d. (n=3). (g) Effects of S1PR3 antagonists (TY52156, 1 μM; CAY10444, 10 μM) and the S1PR2 antagonist (JTE013, 10 μM) on S1P-induced increase in the ALDH-positive cell population. Data represent mean±s.d. (n=3). (h) After transfection with siRNA, expression levels of S1P receptor were examined by qPCR and immunoblotting. Effects of siRNAs againstS1PR3andS1PR2on S1P-induced increase in the ALDH-positive cell population. Data represent mean±s.d. (n=3). Expression levels were normalized to glyceraldehyde 3-phosphate dehydrogenase messenger RNAs. Figure 1: Role of S1PR3 in the ALDH-positive cell population within the MCF-7 cell line. ( a ) Expression levels of S1PR ( S1PR2 and S1PR3 ) in parental or ALDH-positive MCF-7 cells by qPCR. Data represent mean±s.d. ( n =3). ( b ) Representative flow data with ALDH substrate in the presence or absence of S1P (100 nM, 3 days) in MCF-7 cells. Dose-dependent effects of S1P in the proportion of ALDH-positive cell population. Data represent mean±s.d. ( n =3). ( c ) Representative flow data of the SP assay with Hoechst 33342 dye alone or in the presence of reserpine (15 μg ml −1 ). ( d ) Effects of S1P (100 nM) on mammosphere-forming efficiency in MCF-7 cells. The number of mammospheres was microscopically counted and the percentage of mammosphere-forming cells was determined as mammosphere-forming efficiency (%). The scale bar, 100 μm. Data represent mean±s.d. ( n =3). ( e ) Effects of S1P (100 nM) on CD44 + /CD24 − population in MCF-7 cells. ( f ) Effects of S1P (100 nM) on expression of stem cell markers by qPCR. Data represent mean±s.d. ( n =3). ( g ) Effects of S1PR3 antagonists (TY52156, 1 μM; CAY10444, 10 μM) and the S1PR2 antagonist (JTE013, 10 μM) on S1P-induced increase in the ALDH-positive cell population. Data represent mean±s.d. ( n =3). ( h ) After transfection with siRNA, expression levels of S1P receptor were examined by qPCR and immunoblotting. Effects of siRNAs against S1PR3 and S1PR2 on S1P-induced increase in the ALDH-positive cell population. Data represent mean±s.d. ( n =3). Expression levels were normalized to glyceraldehyde 3-phosphate dehydrogenase messenger RNAs. Full size image S1P enhances Notch signalling via S1PR3 Growing evidence suggests many similarities between embryonic stem cells and CSCs [9] ; therefore, we focused on Notch, Hedgehog and Wnt as signalling pathway candidates downstream of the S1PR. Stimulation with S1P induced expression of the Notch target gene Hes1 in MCF-7 cells ( Fig. 2a ) and ALDH-positive MCF-7 cells ( Supplementary Fig. 7a ). Moreover, S1P also induced the Hes1 expression in ALDH-positive A549, LNCaP, U251 and OVCAR-5 cells ( Supplementary Fig. 7b ). S1P-induced Hes1 expression was inhibited by S1PR3 antagonists ( Fig. 2b ). In contrast, the Hedgehog target gene Gli1 , and Wnt target gene Dkk1 were not induced. The effect of S1P on ALDH-positive cell population was inhibited by DAPT, an inhibitor of γ-secretase, which has multiple substrates including Notch, not by the Hedgehog inhibitor cyclopamine and the Wnt inhibitor PNU74654 ( Fig. 2c ; Supplementary Fig. 8 ). Similar effects of DAPT were obtained in MDA-MB-231 cells ( Supplementary Fig. 5d ), A549 cells, LNCaP cells, U251 cells and OVCAR-5 cells ( Supplementary Fig. 6b ). To determine whether S1P has the ability to activate the Notch pathway, we examined cleavage of Notch in MCF-7 cells. Stimulation with S1P produced the Notch intracellular domain (N1ICD) ( Fig. 2d ) and induced activation of the Notch transcriptional reporter CSL -luc ( Fig. 2e ). Because Hes1 expression is dependent on NICD/CSL/MAML complex-mediated gene transcription [22] , we verified whether co-activators were involved in CSCs, using dominant-negative (DN) mutants of CSL, which have been reported to have no ability to bind to DNA [23] . DN-CSL inhibited S1P-induced Hes1 expression and the ALDH-positive cell population ( Fig. 2f ). Similar results were obtained by DN-MAML, which lacks transcriptional activating domain and inhibits NICD-dependent transcriptional activition [24] . To examine which subtype of Notch was involved in CSCs, we overexpressed each type of NICD. Overexpression of N1ICD increased Hes1 expression and the ALDH-positive cell population ( Fig. 2g ). N3ICD also increased the ALDH-positive cell population ( Supplementary Fig. 9a ), while N2ICD and N4ICD had little effect. S1P-induced N1ICD production was inhibited by CAY10444 ( Fig. 2h ); however, S1P did not induce N3ICD production ( Supplementary Fig. 9b ). To further examine the involvement of Notch in CSC, we performed knockdown experiments using Notch1 siRNA. Knockdown of Notch1 inhibited the effect of S1P on ALDH-positive cell population ( Fig. 2i ; Supplementary Fig. 10 ). Taken together, these data suggest crosstalk between S1P and Notch1. To confirm the involvement of S1PR3 in crosstalk, we studied subtype of G proteins coupled to S1PR3. Pertussis toxin (PTX), which inactivates G i protein, abolished S1P-induced Hes1 expression and the ALDH-positive cell population, whereas C3 toxin, which inactivates an effector of G 12/13 Rho, had little effect ( Fig. 2j ). The effects of toxins were confirmed by overexpression of constitutively active (CA) mutants for G i , but not by CA-G 12 ( Fig. 2k ). These data suggest that G i mediates S1P-induced Notch activation via S1PR3. Collectively, S1P has an ability to increase the number of CSCs via Notch signalling in several types of cancer. 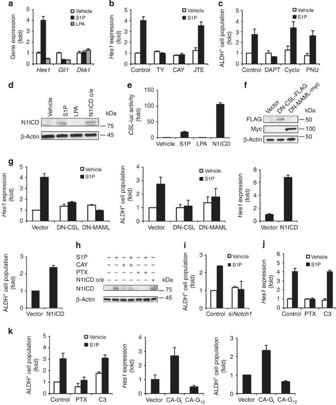Figure 2: Role of Notch signalling in ALDH-positive cell population. (a) After stimulation with S1P (100 nM) or LPA (100 nM) for 24 h, expression levels of the Notch target gene (Hes1), Hedgehog target gene (Gli1) and Wnt target gene (Dkk1) were quantified in MCF-7 cells using qPCR. Data represent mean±s.d. (n=3). (b) Effects of TY52156 (1 μM) or CAY10444 (10 μM) on S1P-inducedHes1expression using qPCR. Data represent mean±s.d. (n=3). (c) Effects of the Notch inhibitor DAPT (5 μM), the Hedgehog inhibitor cyclopamine (10 μM) or the Wnt inhibitor PNU74654 (10 μM) on S1P-induced increase in the ALDH-positive cell population. Data represent mean±s.d. (n=3). (d) Effects of S1P or LPA on N1ICD production by immunoblotting. (e) MCF-7 cells transfected with a reporter plasmid encoding CSL-luc were cultured with or without S1P or LPA and were then analysed by luciferase assays. Data represent mean±s.d. (n=3). (f) Effects of overexpression of Flag-tagged DN-CSL or myc-tagged DN-MAML on S1P-inducedHes1expression and ALDH-positive cell population. Data represent mean±s.d. (n=3). The expression of plasmids was analysed by immunoblotting using tag-specific antibodies. (g) Effects of overexpression of N1ICD onHes1expression and ALDH-positive cell population. Data represent mean±s.d. (n=3). (h) After pretreatment with PTX (0.1 μg ml−1, 24 h) or CAY10444 (10 μM, 30 min), the cells were stimulated with S1P. N1ICD production was analysed by immunoblotting with N1ICD-specific antibodies. (i) Effects of siRNA againstNotch1on S1P-induced increase in the ALDH-positive cell population. Data represent mean±s.d. (n=3). (j) Effects of toxins (PTX, 0.1 μg ml−1; C3 Toxin, 0.1 μg ml−1) on S1P-inducedHes1expression and ALDH-positive cell population. Data represent mean±s.d. (n=3). (k) Effects of overexpression of CA mutants of Gior G12on S1P-inducedHes1expression and ALDH-positive cell population. Data represent mean±s.d. (n=3). Expression levels were normalized to glyceraldehyde 3-phosphate dehydrogenase messenger RNAs. Figure 2: Role of Notch signalling in ALDH-positive cell population. ( a ) After stimulation with S1P (100 nM) or LPA (100 nM) for 24 h, expression levels of the Notch target gene ( Hes1 ), Hedgehog target gene ( Gli1 ) and Wnt target gene ( Dkk1 ) were quantified in MCF-7 cells using qPCR. Data represent mean±s.d. ( n =3). ( b ) Effects of TY52156 (1 μM) or CAY10444 (10 μM) on S1P-induced Hes1 expression using qPCR. Data represent mean±s.d. ( n =3). ( c ) Effects of the Notch inhibitor DAPT (5 μM), the Hedgehog inhibitor cyclopamine (10 μM) or the Wnt inhibitor PNU74654 (10 μM) on S1P-induced increase in the ALDH-positive cell population. Data represent mean±s.d. ( n =3). ( d ) Effects of S1P or LPA on N1ICD production by immunoblotting. ( e ) MCF-7 cells transfected with a reporter plasmid encoding CSL-luc were cultured with or without S1P or LPA and were then analysed by luciferase assays. Data represent mean±s.d. ( n =3). ( f ) Effects of overexpression of Flag-tagged DN-CSL or myc-tagged DN-MAML on S1P-induced Hes1 expression and ALDH-positive cell population. Data represent mean±s.d. ( n =3). The expression of plasmids was analysed by immunoblotting using tag-specific antibodies. ( g ) Effects of overexpression of N1ICD on Hes1 expression and ALDH-positive cell population. Data represent mean±s.d. ( n =3). ( h ) After pretreatment with PTX (0.1 μg ml −1 , 24 h) or CAY10444 (10 μM, 30 min), the cells were stimulated with S1P. N1ICD production was analysed by immunoblotting with N1ICD-specific antibodies. ( i ) Effects of siRNA against Notch1 on S1P-induced increase in the ALDH-positive cell population. Data represent mean±s.d. ( n =3). ( j ) Effects of toxins (PTX, 0.1 μg ml −1 ; C3 Toxin, 0.1 μg ml −1 ) on S1P-induced Hes1 expression and ALDH-positive cell population. Data represent mean±s.d. ( n =3). ( k ) Effects of overexpression of CA mutants of G i or G 12 on S1P-induced Hes1 expression and ALDH-positive cell population. Data represent mean±s.d. ( n =3). Expression levels were normalized to glyceraldehyde 3-phosphate dehydrogenase messenger RNAs. Full size image S1P increases ADAM17 activity without Notch ligands We further investigated the molecular mechanism of crosstalk between S1P and Notch in MCF-7 cells. Notch is generally activated by binding of Notch ligands to Notch and then cleaved by ADAM17 and γ-secretase [25] . Among Notch ligands (Jagged1, 2 and Delta-like ligand (Dll) 1, 3 and 4), Dll3 is not capable to activate Notch signalling in adjacent cells [26] . To examine whether Notch ligands are required for the S1P effect, we examined the expression level of Notch ligands. S1P did not induce expression levels of Notch ligands ( Supplementary Fig. 11a ). Knockdown of Notch ligands did not affect S1P-induced Hes1 expression and ALDH-positive cell population ( Fig. 3a,b ). In contrast to S1P, knockdown of Notch ligands inhibited hypoxia-mimetic agent desferoxamine-induced Hes1 expression. In addition, neutralizing antibodies to Jagged1 inhibited Hes1 induction by soluble Jagged1-Fc, but not S1P-induced Hes1 expression and ALDH-positive cell population ( Supplementary Fig. 11c,d ). Taken together, these data suggest that S1P activates Notch signalling in Notch ligand-independent manner. 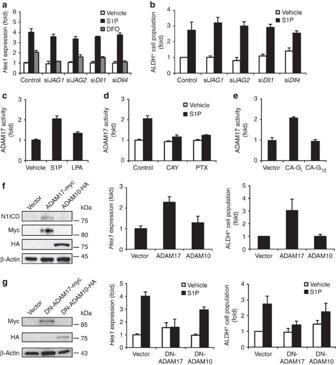Figure 3: S1P increases ALDH-positive cell population without Notch ligands. (a) Effects of siRNA againstJagged1,Jagged2,Dll1andDll4on desferoxamine- or S1P-inducedHes1expression. Data represent mean±s.d. (n=3). (b) Effects of siRNA againstJagged1,Jagged2,Dll1andDll4on S1P-induced increase in ALDH-positive cell population. Data represent mean±s.d. (n=3). (c) Stimulation with S1P (100 nM, 4 h) increased ADAM17 enzyme activity. Data represent mean±s.d. (n=3). (d) S1P-induced ADAM17 activation was inhibited by CAY10444 (10 μM) and PTX (0.1 μg ml−1). Data represent mean±s.d. (n=3). (e) ADAM17 activation was induced by the overexpression of CA-Gi, but not by CA-G12. Data represent mean±s.d. (n=3). (f) Immunoblotting of N1ICD in ADAM17-myc- and ADAM10-HA-overexpressed MCF-7 cells. The expression of plasmids was confirmed using tag-specific antibody. Effects of overexpression of ADAM17 or ADAM10 onHes1expression in MCF-7 cells. Effects of overexpression of ADAM17 or ADAM10 on ALDH-positive cell population in MCF-7 cells. Data represent mean±s.d. (n=3). (g) Effects of DN mutants of ADAM17 or DN-ADAM10 on S1P-inducedHes1expression and the ALDH-positive cell population. Data represent mean±s.d. (n=3). Expression levels were normalized to glyceraldehyde 3-phosphate dehydrogenase messenger RNAs. Figure 3: S1P increases ALDH-positive cell population without Notch ligands. ( a ) Effects of siRNA against Jagged1 , Jagged2 , Dll1 and Dll4 on desferoxamine- or S1P-induced Hes1 expression. Data represent mean±s.d. ( n =3). ( b ) Effects of siRNA against Jagged1 , Jagged2 , Dll1 and Dll4 on S1P-induced increase in ALDH-positive cell population. Data represent mean±s.d. ( n =3). ( c ) Stimulation with S1P (100 nM, 4 h) increased ADAM17 enzyme activity. Data represent mean±s.d. ( n =3). ( d ) S1P-induced ADAM17 activation was inhibited by CAY10444 (10 μM) and PTX (0.1 μg ml −1 ). Data represent mean±s.d. ( n =3). ( e ) ADAM17 activation was induced by the overexpression of CA-G i , but not by CA-G 12 . Data represent mean±s.d. ( n =3). ( f ) Immunoblotting of N1ICD in ADAM17-myc- and ADAM10-HA-overexpressed MCF-7 cells. The expression of plasmids was confirmed using tag-specific antibody. Effects of overexpression of ADAM17 or ADAM10 on Hes1 expression in MCF-7 cells. Effects of overexpression of ADAM17 or ADAM10 on ALDH-positive cell population in MCF-7 cells. Data represent mean±s.d. ( n =3). ( g ) Effects of DN mutants of ADAM17 or DN-ADAM10 on S1P-induced Hes1 expression and the ALDH-positive cell population. Data represent mean±s.d. ( n =3). Expression levels were normalized to glyceraldehyde 3-phosphate dehydrogenase messenger RNAs. Full size image We next studied cleavage enzymes that are responsible for S1P-induced Notch activation. We found that stimulation with S1P increased ADAM17 activity in MCF-7 cells ( Fig. 3c ) and ALDH-positive MCF-7 cells ( Supplementary Fig. 7c ). In addition, S1P also increased γ-secretase activity in MCF-7 cells ( Supplementary Fig. 12a ). CAY10444 and PTX inhibited S1P-induced ADAM17 activation ( Fig. 3d ) and γ-secretase activation ( Supplementary Fig. 12b ). Overexpression of CA-G i also increased both ADAM17 ( Fig. 3e ) and γ-secretase activity ( Supplementary Fig. 12c ). Moreover, we examined whether ADAM17 activation occurred in CSCs. Overexpression of ADAM17 increased N1ICD production, Hes1 expression and the ALDH-positive cell population ( Fig. 3f ). Conversely, DN-ADAM17 (E406A; point mutation at metalloprotease domain) [27] inhibited S1P-induced responses ( Fig. 3g ). Expression of ADAM10 or DN-ADAM10 (E384A; point mutation at metalloprotease domain) [28] had little effect on the CSC signalling pathway. These data suggest that ADAM17 is involved in S1P-induced CSC proliferation. p38MAPK mediates ADAM17 activation by S1P We investigated whether the intracellular domain of ADAM17 plays a role in S1P-induced breast CSC proliferation. ADAM17 activity is regulated by phosphorylation-dependent mechanisms [29] , [30] , [31] ; therefore, we generated ADAM17 mutants with either Thr735 (p38MAPK consensus motif) or Thr761 (Akt consensus motif) replaced by alanine ( Fig. 4a ). Consistent with our data above, S1P induced ADAM17 phosphorylation at Thr735 ( Fig. 4b ). S1P-induced ADAM17 phosphorylation was inhibited by PTX and CAY10444. A mutation at Thr735 decreased ADAM17 phosphorylation through S1P, whereas a mutation at Thr761 had little effect ( Fig. 4c ). In addition, mutation of Thr735 inhibited S1P-induced ADAM17 activation, Hes1 expression and the number of ALDH-positive cell population ( Fig. 4d ). To further confirm the involvement of p38MAPK, we studied the association between p38MAPK and ADAM17. Stimulation with S1P induced a transient phosphorylation of p38MAPK ( Supplementary Fig. 13a ) and an association between p38MAPK and ADAM17 ( Fig. 4e ). Mutation of Thr735 abolished this association ( Fig. 4f ), suggesting that phospho-p38MAPK binds to ADAM17 at Thr735. Treatment with CAY10444 or PTX also inhibited the S1P-induced association between p38MAPK and ADAM17 ( Fig. 4g ). The p38MAPK inhibitor SB203580 inhibited the S1P-induced responses ( Supplementary Fig. 13b–d ). Furthermore, SB203580 inhibited the association between p38MAPK and ADAM17 ( Supplementary Fig. 13f ). In contrast, the PI3-kinase/Akt pathway inhibitor LY294002 had little effect ( Supplementary Fig. 13b–e ). Taken together, these data suggest that p38MAPK-mediated ADAM17 activation is involved in the S1P-induced CSC phenotype. 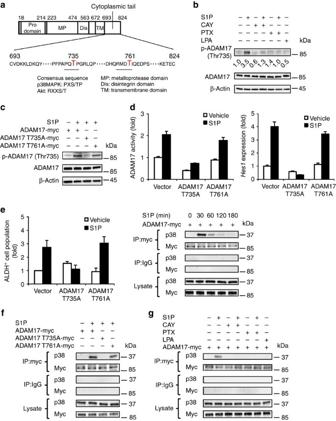Figure 4: S1P-induced ADAM17 activation via p38MAPK. (a) A schematic of the ADAM17 cytoplasmic domain mutants. (b) S1P-induced phosphorylation of ADAM17 at Thr735 was analysed by immunoblotting with a phospho-ADAM17 (Thr735)-specific antibody. (c) MCF-7 cells were transfected with ADAM17-T735A-myc or ADAM17-T761A-myc mutants and were then immunoblotted with phospho-ADAM17 (Thr735)-specific antibodies. (d) Effects of ADAM17-T735A and ADAM17-T761A mutants on S1P-induced ADAM17 activation,Hes1expression and ALDH-positive cell population. Expression levels were normalized to glyceraldehyde 3-phosphate dehydrogenase messenger RNAs. Data represent mean±s.d. (n=3). (e) MCF-7 cells transfected with myc-tagged ADAM17 were either treated or untreated with S1P (100 nM) for the indicated times. The cells were then lysed and subjected immunoprecipitation with myc-specific antibodies, followed by p38MAPK-specific immunoblotting. (f) MCF-7 cells were transfected with myc-tagged ADAM17-T735A or T761A and stimulated with S1P (100 nM) for 30 min. The cells were then lysed and subjected to immunoprecipitation with myc-specific antibodies, followed by p38MAPK-specific immunoblotting. (g) MCF-7 cells transfected with myc-tagged ADAM17 were treated with S1P (100 nM) or LPA (100 nM) for 30 min in the presence or absence of CAY10444 (10 μM) or PTX (0.1 μg ml−1). The cells were lysed and subjected to immunoprecipitation with myc-specific antibodies, followed by p38MAPK-specific immunoblotting. Figure 4: S1P-induced ADAM17 activation via p38MAPK. ( a ) A schematic of the ADAM17 cytoplasmic domain mutants. ( b ) S1P-induced phosphorylation of ADAM17 at Thr735 was analysed by immunoblotting with a phospho-ADAM17 (Thr735)-specific antibody. ( c ) MCF-7 cells were transfected with ADAM17-T735A-myc or ADAM17-T761A-myc mutants and were then immunoblotted with phospho-ADAM17 (Thr735)-specific antibodies. ( d ) Effects of ADAM17-T735A and ADAM17-T761A mutants on S1P-induced ADAM17 activation, Hes1 expression and ALDH-positive cell population. Expression levels were normalized to glyceraldehyde 3-phosphate dehydrogenase messenger RNAs. Data represent mean±s.d. ( n =3). ( e ) MCF-7 cells transfected with myc-tagged ADAM17 were either treated or untreated with S1P (100 nM) for the indicated times. The cells were then lysed and subjected immunoprecipitation with myc-specific antibodies, followed by p38MAPK-specific immunoblotting. ( f ) MCF-7 cells were transfected with myc-tagged ADAM17-T735A or T761A and stimulated with S1P (100 nM) for 30 min. The cells were then lysed and subjected to immunoprecipitation with myc-specific antibodies, followed by p38MAPK-specific immunoblotting. ( g ) MCF-7 cells transfected with myc-tagged ADAM17 were treated with S1P (100 nM) or LPA (100 nM) for 30 min in the presence or absence of CAY10444 (10 μM) or PTX (0.1 μg ml −1 ). The cells were lysed and subjected to immunoprecipitation with myc-specific antibodies, followed by p38MAPK-specific immunoblotting. Full size image SphK1 increases CSCs via S1PR3 S1P is synthesized through SphK-catalyzed phosphorylation of sphingosine [11] , [14] . We next examined whether SphK is involved in breast CSCs. Consistent with previous reports [32] , [33] , overexpressed SphK1 was localized in the cytosol, and SphK2 was mainly localized to the nucleus ( Fig. 5a ). Enzyme activities of SphKs were also confirmed ( Supplementary Fig. 14 ). Overexpression of SphK1 increased the number of ALDH-positive cell population in both MCF-7 ( Fig. 5b ) and MDA-MB-231 cells ( Supplementary Fig. 15 ), whereas SphK2 had little effect. Consistent with the ALDH assay results, ADAM17 activation, N1ICD production and Hes1 expression were induced by SphK1 but not SphK2 ( Fig. 5c ). To determine whether intracellular S1P is involved in the SphK1 effect, we tested the effects of the S1PR3 antagonist on SphK1-induced increases in the ALDH-positive cell population. Pretreatment with CAY10444 inhibited SphK1-induced responses ( Fig. 5d ). S1PR3 shRNAs also inhibited these SphK1-induced responses ( Fig. 5e ). Analysis by qPCR confirmed specific suppression of S1PR3 by these shRNAs ( Fig. 5e ), and treatment with PTX also produced similar results. Recent studies suggest that the ABC transporter mediates oestrogen-induced S1P secretion in MCF-7 cells [34] . To determine whether the ABC transporter is involved with the SphK1 effect, we used siRNAs and a selective inhibitor to inhibit the transporter. An siRNA against ABCC1 inhibited SphK1-induced ADAM17 activation, Hes1 expression and the ALDH-positive cell population ( Supplementary Fig. 16a ). The ABCC1 inhibitor MK571 also produced similar results ( Supplementary Fig. 16b ). In contrast, an siRNA against Spns2 , another S1P transporter [35] , had little effects. These data suggest that S1P produced by SphK1 stimulates S1PR3, and leads to an increase in the number of CSCs. 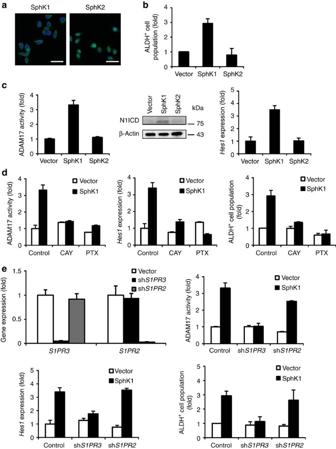Figure 5: Role of SphK1 in ALDH-positive cell population. (a) Expression of SphK in MCF-7 cells. Plasmid vectors encoding FLAG-tagged SphK1, or HA-tagged SphK2 were transfected into MCF-7 cells before SphK protein levels in cells were analysed by immunostaining. The scale bar indicates 20 μm. (b) Effects of SphK1 and SphK2 on the ALDH-positive cell population. Data represent mean±s.d. (n=3). (c) Effects of SphK1 and SphK2 on ADAM17 activity, NICD production, andHes1expression. Data represent mean±s.d. (n=3). (d) Effects of CAY10444 (10 μM) and PTX (0.1 μg ml−1) on the SphK1-induced ADAM17 activity,Hes1expression and ALDH-positive cell population. Data represent mean±s.d. (n=3). (e) Expression level of S1P receptor in shRNA-transduced MCF-7 cells. Effects of shRNAs againstS1PR3andS1PR2on the SphK1-induced ADAM17 activity,Hes1expression and ALDH-positive cell population. Data represent mean±s.d. (n=3). Expression levels were normalized to glyceraldehyde 3-phosphate dehydrogenase messenger RNAs. Figure 5: Role of SphK1 in ALDH-positive cell population. ( a ) Expression of SphK in MCF-7 cells. Plasmid vectors encoding FLAG-tagged SphK1, or HA-tagged SphK2 were transfected into MCF-7 cells before SphK protein levels in cells were analysed by immunostaining. The scale bar indicates 20 μm. ( b ) Effects of SphK1 and SphK2 on the ALDH-positive cell population. Data represent mean±s.d. ( n =3). ( c ) Effects of SphK1 and SphK2 on ADAM17 activity, NICD production, and Hes1 expression. Data represent mean±s.d. ( n =3). ( d ) Effects of CAY10444 (10 μM) and PTX (0.1 μg ml −1 ) on the SphK1-induced ADAM17 activity, Hes1 expression and ALDH-positive cell population. Data represent mean±s.d. ( n =3). ( e ) Expression level of S1P receptor in shRNA-transduced MCF-7 cells. Effects of shRNAs against S1PR3 and S1PR2 on the SphK1-induced ADAM17 activity, Hes1 expression and ALDH-positive cell population. Data represent mean±s.d. ( n =3). Expression levels were normalized to glyceraldehyde 3-phosphate dehydrogenase messenger RNAs. Full size image SphK1 accelerates tumour formation of CSCs via S1PR3 Since S1P is easily degraded by S1P lyase or phosphatases, we next studied tumorigenicity using SphK1- or SphK2-overexpressing CSCs in MCF-7 cells. Almost all nude mice injected with SphK1-overexpressing ALDH-positive cells developed tumours within 6 weeks. Tumour formation was inefficient in the mice injected with vector- or SphK2-overexpressing ALDH-positive cells ( Fig. 6a,b ). Tumour sizes from SphK1-overexpressing ALDH-positive cells were bigger than those from vector- or SphK2-overexpressing ALDH-positive cells ( Fig. 6c,d ). Histological analysis indicated that tumours derived from the ALDH-positive cells and the SphK1-overexpressing ALDH-positive cells had similar morphologies ( Fig. 6e ). To examine the proportion of ALDH-positive cells in xenografted tumour samples, we conducted double staining using ALDH assays and human-specific antibodies to TRA-1-85 ( Supplementary Fig. 17 ). The increase in the proportion of ALDH-positive cells in the tumour paralleled the in vitro results, suggesting a stem cell hierarchy ( Fig. 6f ). Histological analysis and double staining suggest that it is unlikely that the enhanced incidence of tumour formation by expression of SphK1 was due to cell differentiation. To examine whether S1PR3 and ALDH1 were co-expressed in the same cell, we performed double staining of ALDH1 and S1PR3 using xenografted tumour section ( Supplementary Fig. 18 ). The number of ALDH1- and S1PR3 double-positive cells was increased in tumours derived from the SphK1-overexpressing ALDH-positive cells, compared with control and SphK2-overexpressing ALDH-positive cells. In addition, knockdown of S1PR3 significantly inhibited the tumorigenicity of SphK1-overexpressing ALDH-positive cells, whereas knockdown of S1PR2 had little effect ( Fig. 6g ). Furthermore, chronic administration of the S1PR3 antagonist TY52156 significantly inhibited the tumorigenicity of SphK1-overexpressing ALDH-positive cells ( Fig. 6h ). Taken together, both in vitro and in vivo results suggest that enhanced expression of SphK1 accelerated tumour formation of CSCs via S1PR3. 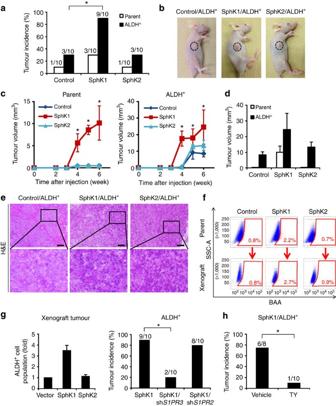Figure 6: SphK1 increases CSC-mediated tumour formation in a mouse xenograft model. (a) Balb/c nude mice were subcutaneously injected with 1 × 105vector- or SphK-transfected MCF-7 cells. Tumour formation was indicated by tumours/injections at 6 weeks post injection. ThePvalue was calculated using the Fisher's exact test. Bonferroni correction was applied for multiple comparisons. *P<0.05 versus control. (b) Photographs of representative nude mice transplanted with ALDH-positive cells, SphK1-overexpressing ALDH-positive cells and SphK2-overexpressing ALDH-positive cells. (c) Tumour growth curves in the nude mice injected with parent or ALDH-positive cells. Tumour volume is presented as the mean±s.d. (n=10). Kruskal–Wallis test, followed by the Steel–Dwass was used to determine significance. *P<0.05 versus control. (d) Tumour volumes at 6 weeks post injection. Data represent mean±s.d. (n=10). (e) Hematoxylin/eosin (H&E)-stained sections of tumour xenografts derived from vector-, SphK1-, and SphK2-overexpressing ALDH-positive cells. Scale bar, 100 μm. (f) Representative flow cytometry analysis of ALDH activity in the xenograft tumours derived from vector-, SphK1-, and SphK2-overexpressing ALDH-positive cells. The graph indicates ALDH-positive cell population in xenograft tumours. Data represent mean±s.d. (n=3). ALDH-positive cells were able to regenerate the phenotypic heterogeneity in the xenograft tumours of nude mice. (g) Balb/c nude mice were subcutaneously injected with 1 × 105vector-,S1PR3- orS1PR2-knockdown cells from SphK1-overexpressing ALDH-positive cells. Tumor formation was indicated by tumours/injections at 6 weeks post injection. ThePvalue was calculated using the Fisher's exact test. Bonferroni correction was applied for multiple comparisons. *P<0.05 versus control. (h) TY52156 or vehicle was inserted in subcutaneously implanted Alzet osmotic pumps before injection of 1 × 105SphK1-overexpressing ALDH-positive cells. Tumour formation was indicated by tumours/injections at 6 weeks post injection. ThePvalue was calculated using the Fisher's exact test. *P<0.05 versus control. Figure 6: SphK1 increases CSC-mediated tumour formation in a mouse xenograft model. ( a ) Balb/c nude mice were subcutaneously injected with 1 × 10 5 vector- or SphK-transfected MCF-7 cells. Tumour formation was indicated by tumours/injections at 6 weeks post injection. The P value was calculated using the Fisher's exact test. Bonferroni correction was applied for multiple comparisons. * P <0.05 versus control. ( b ) Photographs of representative nude mice transplanted with ALDH-positive cells, SphK1-overexpressing ALDH-positive cells and SphK2-overexpressing ALDH-positive cells. ( c ) Tumour growth curves in the nude mice injected with parent or ALDH-positive cells. Tumour volume is presented as the mean±s.d. ( n =10). Kruskal–Wallis test, followed by the Steel–Dwass was used to determine significance. * P <0.05 versus control. ( d ) Tumour volumes at 6 weeks post injection. Data represent mean±s.d. ( n =10). ( e ) Hematoxylin/eosin (H&E)-stained sections of tumour xenografts derived from vector-, SphK1-, and SphK2-overexpressing ALDH-positive cells. Scale bar, 100 μm. ( f ) Representative flow cytometry analysis of ALDH activity in the xenograft tumours derived from vector-, SphK1-, and SphK2-overexpressing ALDH-positive cells. The graph indicates ALDH-positive cell population in xenograft tumours. Data represent mean±s.d. ( n =3). ALDH-positive cells were able to regenerate the phenotypic heterogeneity in the xenograft tumours of nude mice. ( g ) Balb/c nude mice were subcutaneously injected with 1 × 10 5 vector-, S1PR3 - or S1PR2 -knockdown cells from SphK1-overexpressing ALDH-positive cells. Tumor formation was indicated by tumours/injections at 6 weeks post injection. The P value was calculated using the Fisher's exact test. Bonferroni correction was applied for multiple comparisons. * P <0.05 versus control. ( h ) TY52156 or vehicle was inserted in subcutaneously implanted Alzet osmotic pumps before injection of 1 × 10 5 SphK1-overexpressing ALDH-positive cells. Tumour formation was indicated by tumours/injections at 6 weeks post injection. The P value was calculated using the Fisher's exact test. * P <0.05 versus control. Full size image Patient-derived CSCs contain SphK1 + /ALDH1 + cells We further extended our observations to primary cell culture. To examine S1PR3 expression level in breast CSCs, we performed qPCR using secondary mammospheres from patient-derived tumour [8] ( Supplementary Table 1 ). Similar to MCF-7 cells, S1PR3 was highly expressed in ALDH-positive cells derived from breast cancer patient ( Fig. 7a ). In addition, we evaluated whether there were co-expressions of SphK1/ALDH1 or S1PR3/ALDH1 in breast CSCs by immunochemistry. Double staining demonstrated that these patient samples contained SphK1- and ALDH1 double-positive cells or S1PR3- and ALDH1 double-positive cells ( Fig. 7b,c ). We further evaluated whether SphK1, ADAM17 and N1ICD were co-expressed in the same cell. As a result, patient-derived tumour cells contained triple-positive cells ( Fig. 7d ). These data suggest that SphK1/S1PR3/Notch signalling is present in CSCs derived from breast cancer patient. 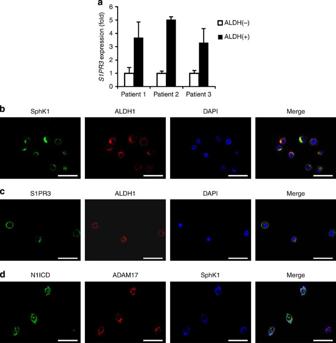Figure 7: SphK1-positive CSCs in human breast cancers. (a)S1PR3expression in the ALDH-negative or ALDH-positive patient-derived cells by qPCR. Expression levels were normalized to glyceraldehyde 3-phosphate dehydrogenase messenger RNAs. Data represent mean±s.d. (n=3). (b) Double immunostaining of SphK1 (green) and ALDH1 (red) in patient-derived tumour cells. Nuclei were counterstained by DAPI (blue). (c) Double immunostaining of S1PR3 (green) and ALDH1 (red) in patient-derived tumour cells. Nuclei were counterstained by DAPI (blue). (d) Triple immunostaining of N1ICD (green), ADAM17 (red) and SphK1 (blue) in patient-derived tumour cells. Scale bar, 20 μm. Figure 7: SphK1-positive CSCs in human breast cancers. ( a ) S1PR3 expression in the ALDH-negative or ALDH-positive patient-derived cells by qPCR. Expression levels were normalized to glyceraldehyde 3-phosphate dehydrogenase messenger RNAs. Data represent mean±s.d. ( n =3). ( b ) Double immunostaining of SphK1 (green) and ALDH1 (red) in patient-derived tumour cells. Nuclei were counterstained by DAPI (blue). ( c ) Double immunostaining of S1PR3 (green) and ALDH1 (red) in patient-derived tumour cells. Nuclei were counterstained by DAPI (blue). ( d ) Triple immunostaining of N1ICD (green), ADAM17 (red) and SphK1 (blue) in patient-derived tumour cells. Scale bar, 20 μm. Full size image In the present study, we used ALDH assays to identify regulators in CSCs, and determined that S1P/S1PR3 signalling and subsequent Notch activation resulted in an increase in the CSCs in several types of cancer ( Fig. 8 ). S1PR3 antagonist inhibited the tumorigenicity of SphK1-overexpressed breast CSCs. Furthermore, breast cancer patient-derived CSCs contained SphK1 + /ALDH1 + cells or S1PR3 + /ALDH1 + cells. The findings presented here broaden our understanding of the role of lipids in CSC biology, and have significant clinical implications. 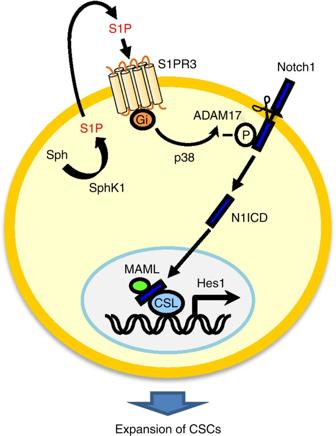Figure 8: A working model for the functions of SphK/S1P/S1PR3 in CSC regulation. S1P produced by SphK1 stimulates S1PR3 and subsequently activates Notch signaling in a Notch ligand-independent manner. Activation of S1P signaling pathway leads to expansion of CSCs. Figure 8: A working model for the functions of SphK/S1P/S1PR3 in CSC regulation. S1P produced by SphK1 stimulates S1PR3 and subsequently activates Notch signaling in a Notch ligand-independent manner. Activation of S1P signaling pathway leads to expansion of CSCs. Full size image We found that S1P has the ability to induce proliferation of several types of CSCs, as stimulation with S1P activates Notch signalling, a key stem cell pathway. As such, S1P might have various roles in stem/progenitor cells. Indeed, S1P has been shown to maintain self-renewal of human embryonic stem cells in cooperation with platelet-derived growth factor [36] . Human-induced pluripotent stem cells have also been shown to express S1PR3 messenger RNAs, although their biological effects in induced pluripotent stem cells are yet to be elucidated [37] . We postulate that S1P might have self-renewal properties, and play a key role in stem cell regulation. We also identified S1P-induced Notch activation without Notch ligands. Consistent with our observations, previous studies have shown that ADAM17 mediates ligand-independent Notch activation, while ADAM10 is ligand dependent [38] , [39] . Another study has shown that soluble form of Jagged1 activates Notch signalling without cell–cell contact [40] . Furthermore, a recent study showed that multiple GPCRs, including the S1PR, resulted in shedding of TGFα via ADAM17 activation in HEK293 cells [41] . Within the S1PR family, S1PR3 has higher intrinsic activity for shedding. These data strongly support a signalling pathway between the S1PR and ADAM17 activation in Notch ligands-independent manner. Further studies should be conducted looking at how the Notch system induces CSC phenotypes in breast cancer. Our data demonstrate an essential cell autonomous role of Notch1 in breast CSCs expansion. Harrison et al . [42] has reported that Notch4 also affects breast CSCs. They performed knockdown of Notch paralog (Notch1 and Notch4) using both ESA + /CD44 + /CD24 low and mammosphere prepared from MCF-7 cells, although Notch ICD overexpression was not examined. Notch1 knockdown reduced only mammosphere population, whereas Notch4 knockdown reduced both ESA + /CD44 + /CD24 low and mammosphere populations (as shown in Figs 3a and 4b ). Because Ginestier et al . [4] have already reported that two stem-like cell populations defined by ALDH positive and CD44 + /CD24 − /lin − were not identical, there is a possibility that discrepancy between our present data and Harrison’s report is caused by the differences of cell populations used in the experiments. Thus, Notch paralog possibly plays a role in regulation in different stem cell population. Our clinical samples suggest the crosstalk between Sphk1-S1P-S1PR3 and Notch signalling by co-localization of the components for the crosstalk machinery. Similar observations were obtained using xenografted tumour samples in nude mice. SphK1 has been already shown to be upregulated in patients with breast cancer [43] , and its expression correlates with cancer progression and poor prognosis [43] , [44] , [45] . In addition, S1PR3 is the most highly expressed S1PR in breast cancer cells [46] . Thus, our data provide a potential explanation for significance of Sphk1-S1PR3-Notch axis in breast cancer. Targeting Notch has been expected to facilitate tumour regression [47] . Although several types of Notch inhibitors are quite effective in preclinical models [21] , [48] , [49] , none of the clinical trials conducted so far has examined effectiveness [50] . This prompts us to encourage efforts to explore alternative/additional approaches for targeting Notch. Our evidence suggests that Notch1 is involved in the S1P-induced CSC phenotype. Because lipid signalling acts upstream of the Notch, S1PR3 could be a promising target for various cancer. Indeed, TY52156 inhibited the tumorigenicity of SphK1-overexpressing breast CSCs ( Fig. 6 ). Although several S1PR antagonists are currently available [14] , few have been tested in clinical trials. The feasibility of S1PR3 antagonists in cancer remains to be determined. In conclusion, the identification of S1P-derived CSC phenotype is required for continuous tumour growth, and points to potential culprits of tumour formation in patients. In the future, it might be possible to establish specific treatments that reduce tumorigenesis by targeting ‘stemness’ in cancer. Thus, efforts should be made to develop drugs capable of inhibiting CSC self-renewal and expansion by S1PR3. Materials Antibodies to p38MAPK (#9212), phospho-p38MAPK (#9211), Akt (#9272), phospho-Akt (#9271), Notch1 (#4380), N1ICD (#2421) and Notch3 (#2889) were from Cell Signaling Technology. Antibodies to HA (#H6908), FLAG (M2) (#F1804), myc (#C3956), β-actin (#A5441) and ADAM17 (phospho-Thr735) (#SAB4504073) were from Sigma-Aldrich. Antibody to ADAM17 (#AB19027) was from Millipore. Antibody to APC-conjugated TRA-1-85 (#FAB3195A) was from R&D Systems. Antibody to SphK1 (#AP7237c) was from Abgent. Antibody to ALDH1 (#611194), FITC mouse anti-human CD44 (#555478), PE mouse anti-human CD24 (#555428), FITC mouse IgG2b κ isotype control (#555742) and PE mouse IgG2a κ isotype control (#555574) were from BD Biosciences. Antibodies to S1PR2 (#sc-25491), S1PR3 (#sc-30024) and Spns2 (#130102) were from Santa Cruz Biotechnology. Antibody to SphK1 (#ab46719), ADAM17 (#ab57484), activated Notch1 (#ab8925) and ABCC1 (#ab3368) were from Abcam. Antibody to Alexa488-conjugated anti-rabbit IgG (#A11034) and Alexa555-conjugated anti-mouse IgG (#A21424) were from Invitrogen. S1P, dihydro-S1P, DAPT, SB203580, 5-Fluorouracil and doxorubicin were from Enzo Life Sciences. CAY10444, JTE013, MK571, LY294002, cyclopamine were from Cayman Chemicals. LPA was from Avanti Polar Lipids. Jagged1-Fc, Sonic hedgehog and Wnt3a were from R&D Systems. Botulinum C3 enzyme was from Bio Academia. PTX were from Wako Pure Chemical (Osaka, Japan). Hoechst, reserpine, DFO and PNU74654 were from Sigma-Aldrich, while N,N′-bis(4-chlorophenyl)-3,3-dimethyl-2-oxobutanehydrazonamide (TY52156) was synthesized. All other reagents were of analytical grade and obtained from commercial sources. Cell culture MCF-7 cells (American Type Culture Collection), MDA-MB-231 cells (American Type Culture Collection), A549 cells (European Collection of Cell Cultures) and LNCaP cells (European Collection of Cell Cultures), U251 cells (Japanese Collection of Research Biosources) were cultured in Dulbecco’s modified Eagle’s medium (DMEM; Sigma-Aldrich) supplemented with 10% heat-inactivated fetal bovine serum (FBS; Biological Industries), 100 U ml −1 penicillin and 100 μg ml −1 streptomycin (Gibco BRL). OVCAR-5 cells was cultured in RPMI1640 (Sigma-Aldrich) supplemented with 10% heat-inactivated FBS (Biological Industries), 100 U ml −1 penicillin and 100 μg ml −1 streptomycin (Gibco BRL). Plasmid constructs and reporter assays Plasmids encoding SphK1, SphK2, DN-CSL, DN-MAML, N1ICD, ADAM10 and 12xCSL-luc were kindly provided from Drs Stuart M. Pitson (University of Adelaide), Taro Okada (Kobe University), Aly Karsan (British Columbia Cancer Research Centre), Anthony J. Capobianco (University of Pennsylvania), Spyros Artavanis-Tsakonas (Harvard Medical School), Stefan Lichtenthaler (Ludvig Maximilians University) and Lothar J. Strobl (German Research Center for Environmental Health), respectively. Plasmids encoding N2ICD, N3ICD and N4ICD were kindly provided by Dr Michael J. Hendzel (University of Alberta). Plasmids encoding ADAM17 and DN-ADAM17 were kindly provided by Dr Rik Derynck (University of California, San Francisco). Plasmids encoding CA-G i and CA-G 12 were kindly provided by Dr J. Silvio Gutkind (National Institutes of Health). Plasmids encoding the ADAM17 mutants T735A and T761A were generated by QuikChange Site-Directed Mutagenesis (Stratagene) using pRK5-ADAM17-myc. A plasmid encoding the ADAM10 mutant E384A (DN-ADAM10) was generated by QuikChange Site-Directed Mutagenesis using peak-12-ADAM10-HA. Coding DNA sequences were verified by DNA sequencing. Transfections were conducted with FuGENE HD transfection reagent (Promega). Luciferase activity was assayed 24 h after transfection with 12xCSL-luc using the Glo Luciferase Assay Kit (Promega). Microarray analysis Total RNAs were isolated by Trizol (Invitrogen) and then purified using an RNeasy Mini Kit (Qiagen). Affymetrix Genome U133A gene chips (Affymetrix) were used to examine gene expression patterns according to the manufacturer’s instruction. Genes upregulated more than twofold are shown in Supplementary Data 1 . ALDH assays The ALDEFLUOR kit (Stem Cell Technologies) was used to detect CSC populations with high ALDH enzyme activity according to the manufacture’s instruction [18] . The cells were plated at a density of 3 × 10 5 cells in 100 mm culture dishes. After serum deprivation for 3 days, cells were suspended at a concentration of 1 × 10 6 cells ml −1 in ALDH assay buffer containing the ALDH substrate BAAA (1 μM) and incubated for 30 min at 37 °C. As a negative control, cells were treated with diethylaminobenzaldehyde (15 μM), a specific ALDH inhibitor. A FACS Aria II cell sorter (BD Biosciences) was used to measure the ALDH-positive cell population. Mammosphere-forming assays MCF-7 cells were plated as single cells on ultralow attachment 6-well plates (Corning) at a concentration of 10,000 cells ml −1 in serum-free DMEM supplemented with N 2 supplement (Gibco) and 20 ng ml −1 basic Fibroblast Growth Factor (R&D Systems). After 4 days, the number of mammospheres was microscopically counted and the percentage of mammosphere-forming cells was determined as mammosphere-forming efficiency (%) [7] . SP assays Cells were collected and suspended in prewarmed DMEM containing 2% FBS and 2 mM HEPES buffer. Hoechst 33342 dye (Sigma-Aldrich) was then added to a final concentration of 5 μg ml −1 , and the mixture was incubated with intermittent shaking for 60 min at 37 °C in the presence or absence of reserpine (15 μg ml −1 ; Sigma-Aldrich). Cells were then resuspended in ice-cold phosphate-buffered saline (PBS) containing 2% FBS, and analysed with a FACS Aria II cell sorter (BD Biosciences). CD44 + /CD24 − cell population Cells were resuspended in PBS containing 5% FBS and incubated with FITC mouse anti-human CD44 (#555478, 1:5) and PE mouse anti-human CD24 (#555428, 1:5) for 15 min at 4 °C. FITC mouse IgG2b κ isotype control (#555742, 1:5) and PE mouse IgG2a κ isotype control (#555574, 1:5) were used as negative control. Analysis was performed using a FACS Aria II cell sorter (BD Biosciences). Cell viability assays MCF-7 cells and sorted ALDH-positive cells were plated onto 96-well plates at a density of 5,000 cells well −1 . After overnight culture, cells were treated with 100 μM 5-Fluorouracil or 10 μM doxorubicin. After 72 h, MTS assays were performed, according to the manufacturer’s instruction (Promega). qPCR assays Total RNA was isolated from MCF-7 cells using Trizol (Invitrogen), according to the manufacturer’s instructions. The qPCR assays were conducted with the aid of a QuantiTect SYBR Green RT-PCR Kit (Qiagen) and an ABI PRISM 7900HT sequence detection system (Applied Biosystems). The relative changes in transcript levels for each sample were determined by normalizing to glyceraldehyde 3-phosphate dehydrogenase mRNA levels. Primer sequences used for qPCR analysis are shown in Supplementary Table 2 . Reverse transcription PCR analysis of S1PRs Total RNA was isolated from MCF-7 cells using Trizol, according to the manufacturer’s instructions. A SuperScript III Fast-Strand Synthesis System (Invitrogen) was used for reverse transcription synthesis of cDNAs. PCR amplification was performed with PrimeStar HS DNA polymerase (Takara) using GeneAmp PCR System 9700 (Applied Biosystems). The cycling conditions were as follows: 1 min at 95 °C, 40 cycles of 30 s at 95 °C, 30 s at 54–66 °C, 1 min at 72 °C, following 7 min at 72 °C. Primer sequences used for reverse transcription PCR analysis are shown in Supplementary Table 2 . Transient RNA interference Double-strand RNA oligonucleotides (siRNAs) against S1PR3 , S1PR2 and appropriate control scrambled siRNA were from Santa Cruz Biotechnology. The siRNAs against Notch1 , ABCC1 and Spns2 were from Invitrogen. The siRNAs were transfected into MCF-7 cells using RNAiMax (Invitrogen) according to the manufacturer’s recommendations. Stable knockdown by lentiviral shRNA transduction For stable gene silencing of S1PR3 or S1PR2 , specific shRNA MISSION lentiviruses (Sigma-Aldrich) were transduced into cells. The target sequence was 5′- CCGGGATCCTCTACGCACGCATCTACTCGAGTAGATGCGTGCGTAGAGGATCTTTTTG -3′ for sh S1PR3 and 5′- CCGGACTTTACCACCTGGTACAAAGCTCGAGCTTTGTACCAGGTGGTAAAGTTTTTTG -3′ for sh S1PR2 . The transduced cells were selected in growth medium containing 1.5 μg ml −1 puromycin (Sigma-Aldrich). Immunoblot analysis Cells were lysed in Cell Lysis Buffer (Cell Signaling Technology) on ice for 30 min. Lysates were subjected to sodium dodecyl sulphate polyacrylamide gel electrophoresis and transferred to Immobilon-P Transfer Membrane (Millipore). Membranes were blocked with 5% (w/v) bovine serum albumin in Tris-buffered saline containing 0.1% Tween-20 (TBST) and incubated with primary antibodies overnight at 4 °C. Membranes were then incubated with horseradish peroxidase-conjugated secondary antibodies (Cell Signaling Technology, 1:2,000) for 1 h at room temperature and detected using ECL Prime Western Blotting Detection Reagent (GE Healthcare). Images were acquired using a LAS-3000 Imager (Fujifilm). The density of each band was quantified using an image analyser (Multi Gauge software, Fujifilm). The primary antibodies used were S1PR3 (#sc-30024, 1:2,000), S1PR2 (#sc-25491, 1:1,000), Notch1 (#4380, 1:1,000), N1ICD (#2421, 1:1,000), Notch3 (#2889, 1:1,000), FLAG (#F1804, 1:1,000), myc (#C3956, 1:5,000), HA (#H6908, 1:1,000), phospho-ADAM17 (#SAB4504073, 1:1,000), ADAM17 (#AB19027, 1:1,000), phospho-p38MAPK (#9211, 1:1,000), p38MAPK (#9212, 1:1,000), phospho-Akt (#9271, 1:1,000), Akt (#9272, 1:1,000), SphK1 (#AP7237c, 1:500), SphK2 (a gift from Dr T. Okada at Kobe University, 1:3,000), ABCC1 (#ab3368, 1:1,000), Spns2 (#sc-130102, 1:1,000) and β-actin (#A5441, 1:10,000). Original immunoblots are shown in Supplementary Fig. 19 . Immunocytochemistry SphK-overexpressing MCF-7 cells and mammosphere cells were plated on glass coverslips. Cells were fixed with 4% paraformaldehyde and permeabilized with 0.2% Triton X-100. Coverslips were blocked with 5% FBS and incubated overnight at 4 °C with primary antibodies that recognized FLAG (#F1804, 1:500), HA (#H6908, 1:120), SphK1 (#ab46719, 1:50), S1PR3 (#sc-30024, 1:50), ALDH1 (#611194, 1:100). ADAM17 (#ab57484, 1:300) and activated Notch1 (#ab8925, 1:200). After rinsing with PBS, coverslips were incubated for 1 h at room temperature with Alexa488-conjugated (#A11034, 1:200) or Alexa555-conjugated (#A21424, 1:200) secondary antibody. In the case of triple staining of Sphk1, ALDH1 and N1ICD, antibody to SphK1 was labelled with AMCA conjugation kit (Abcam). After rinsing with PBS, coverslips were incubated with AMCA-conjugated SphK1 antibody (1:100) for 1.5 h. Nuclei were counterstained with DAPI (Nacalai Tesque). Fluorescence images were obtained using a Nikon A1 confocal microscope (Nikon). Immunoprecipitation assay Immunoprecipitation was conducted as previously reported with slight modifications [51] . MCF-7 cells were transfected with myc-tagged ADAM17. At 48 h after transfection, cells were lysed in lysis buffer (20 mM Tris–HCl pH 7.4, 200 mM NaCl, 0.1% NP-40, 10 mM NaF, 1 mM Na 3 VO 4 and complete mini protease inhibitor cocktail (Roche Applied Sciences)). Lysates (100 μg) were incubated with myc-specific polyclonal antibody (#C3956, 1 μg) or normal rabbit IgG (#PM035, MBL, 1 μg) overnight at 4 °C. Subsequently, Protein G Sepharose (Amersham Pharmacia Biotech) was added to the mixture and incubated for an additional 2 h at 4 °C. Beads were washed with lysis buffer and immunoprecipitated proteins analysed by immunoblotting using a p38MAPK-specific polyclonal antibody (#9212) and a myc-specific polyclonal antibody (#C3956). ADAM17 activity ADAM17 activity was measured using a SensoLyte 520 ADAM17 Activity Assay Kit (ANASPEC) according to the manufacture’s instruction [52] . MCF-7 cells were scraped in PBS containing a complete mini protease inhibitor cocktail and lysed using five cycles of freeze–thawing. Lysed cells were centrifuged at 20,000 g for 15 min and pelleted membranes resuspended with assay buffer. Approximately 15 μg of proteins were mixed with substrate for 30 min and fluorescence intensity was measured using a Wallac1420ARVO fluoroscan (Perkin Elmer), with excitation at 490 nm and emission at 520 nm. γ-secretase activity The activity of γ-secretase was measured using a specific fluorogenic substrate assay [53] . Cells were collected in cell lysis buffer containing (20 mM HEPES pH 7.0, 150 mM KCl, 2 mM EDTA, 1% (3-cholamidopropyl) dimethylammonio]-2-hydroxy-1-propanesulfonate (CHAPSO; Dojindo Laboratories), and complete Mini, EDTA-free protease inhibitor cocktail (Roche)). Lysates were centrifuged at 10,000 g for 1 min at 4 °C to remove nuclei and large cell debris. Approximately 5 μg of protein was added to each well of a white 96-well polystyrene microplate (Packard) and an equal volume of assay buffer (50 mM Tris–HCl (pH 6.8), 2 mM EDTA, and 0.25% (3-cholamidopropyl) dimethylammonio]-2-hydroxy-1-propanesulfonate (w/v)) added. 10 μM fluorogenic γ-secretase substrate (Peptide) was added to the plate and samples incubated at 37 °C for 4 h in the dark. Fluorescence intensity was measured using a Wallac1420ARVO fluoroscan (Perkin Elmer) with excitation at 355 nm and emission at 460 nm. SphK activity SphK activity was measured using omega-(7-nitro-2-1,3-benzoxadiazol-4-yl)- D -erythro-sphingosine-labelled fluorescent substrate [54] . Cells were lysed with a single freeze–thaw cycle in 50 mM HEPES (pH 7.4), 10 mM KCl, 15 mM MgCl 2 , 0.1% Triton X-100, 20% glycerol, 2 mM orthovanadate, 2 mM dithiothreitol, 10 mM NaF, 1 mM deoxypyridoxine and complete Mini, EDTA-free protease inhibitor cocktail (Roche). The lysate was cleared by centrifuging at 20,000 g for 15 min at 4 °C. SphK1 activity was measured in 50 mM HEPES (pH 7.4), 15 mM MgCl 2 , 0.5% Triton X-100, 10% glycerol, 5 mM NaF, 1 mM deoxypyridoxine, 2 mM ATP and 10 μM NBD-sphingosine (Avanti Polar Lipids). SphK2 activity was measured in 50 mM HEPES (pH 7.4), 15 mM MgCl 2 , 0.5 M KCl, 10% glycerol, 5 mM NaF, 1 mM deoxypyridoxine, 2 mM ATP and 10 μM NBD- sphingosine. Reactions were started with the addition of 5 μg of lysate protein and incubated for 4 h at room temperature. Reactions were extracted with the addition of 1 M potassium phosphate (pH 8.5), followed by chloroform/methanol (2:1), then cleared at 15,000 g for 1 min. The upper aqueous layer was placed into the wells of white 96-well polystyrene microplates (Packard). Fluorescence intensity was measured with a Wallac1420ARVO fluoroscan (Perkin Elmer) with excitation at 485 nm and emission at 535 nm. Tumorigenicity assay The animal study protocol was reviewed and approved by the animal care and use committee of the institute. Six-week-old female Balb/c nude mice (CLEA Japan) were used in these studies and were given injections of 17-β-estradiol (Sigma-Aldrich) dissolved in pure sesame oil (0.1 mg 0.05 ml −1 sesame oil per mouse, subcutaneously) 1 day before tumour inoculation, and at weekly intervals, according to a previously reported protocol with slight modifications [55] . The ALDH-positive cell population was sorted by FACS (BD Aria II) and suspended in PBS mixed with an equal volume of Matrigel (BD Biosciences). Mice were given bilateral subcutaneous injections of 1 × 10 5 (0.1 ml) cells. Tumour growth was monitored for 6 weeks and analysed. Tumour volume was determined using the formula: V =½ × larger diameter × (smaller diameter) 2 . For the immunohistochemistry, paraffin-embedded sections of breast tumours from xenografts were deparaffinized in xylene and rehydrated in graded alcohol. Antigen retrieval was conducted three times by microwaving the slides in 0.01 M citrate buffer (pH 6.0) for 5 min. Sections were blocked with 5% FBS and incubated for 1.5 h with primary antibodies that recognized S1PR3 (#sc-30024, 1:50) and ALDH1 (#611194, 1:100). After rinsing with PBS, coverslips were incubated for 1 h at room temperature with Alexa488-conjugated (#A11034, 1:200) or Alexa555-conjugated (#A21424, 1:200) secondary antibody. Nuclei were counterstained with DAPI (Nacalai Tesque). Fluorescence images were obtained using a Biorevo BZ-9000 (Keyence). The number of S1PR3- and ALDH1 double-positive cells was counted in five fields [56] . For the hierarchy assay, the xenografts were collected after 6 weeks, dissociated into single cells and TRA-1-85-positive cells analysed using the ALDH assays [57] . Single cells were suspended in ALDH assay buffer containing the BAAA (1 μM) and incubated 30 min at 37 °C. The cells were resuspended in ALDH assay buffer for subsequent staining with the APC-conjugated TRA-1-85 antibody (#FAB3195A, 1:10), which recognizes human cells and thereby allows their discrimination from mouse cells. After incubation for 30 min and following centrifugation, the cells were resuspended in ALDH assay buffer containing 7-AAD (BD Bioscience, #559925) and analysed with a FACS Aria II cell sorter (BD Bioscience). For the chronic administration, TY52156 (167 mg ml −1 in a 1:1 mixture of DMSO and PEG400) was inserted in subcutaneously implanted Alzet osmotic pumps (Cupertino), designed to release TY52156 continuously (at about 25 μg h −1 ) for 6 weeks. Mammosphere formation from primary cells Mammosphere formation using primary cells (Celprogen) was performed [7] , [8] . The cells were plated as single cells in ultralow attachment dishes (Corning) at a density of 20,000 viable cells ml −1 in mammary epithelial growth medium for 7 days. To make secondary mammospheres, primary mammospheres were collected by gentle centrifugation (200 g ), dissociated enzymatically (10 min in 0.05% trypsin–EDTA) and mechanically (pipetting with yellow tips) into a single-cell suspension. The cells obtained from dissociation were then seeded in ultralow attachment dishes in mammary epithelial growth medium again. Statistical analysis Results are shown as mean±s.d. For tumour incidence, the P value was calculated using the Fisher's exact test ( Fig. 6a,g,h ). Bonferroni correction was applied for multiple comparisons ( Fig. 6a,g ). For tumour volume, the P value was calculated using the Kruskal–Wallis test, followed by post hoc Steel–Dwass's multiple comparison test ( Fig. 6c ). Differences at P <0.05 were considered to be significant. Statistical analyses were performed using Excel 2010 with the add-in software. How to cite this article: Hirata, N. et al . Sphingosine-1 phosphate promotes expansion of cancer stem cells via S1PR3 by a ligand-independent Notch activation. Nat. Commun. 5:4806 doi: 10.1038/ncomms5806 (2014). Accession codes : Microarray data have been deposited in the NCBI Gene Expression Omnibus database under accession codes GSE59653 .